Assembly kinetics determine the architecture of α-actinin crosslinked F-actin networks The actin cytoskeleton is organized into diverse meshworks and bundles that support many aspects of cell physiology. Understanding the self-assembly of these actin-based structures is essential for developing predictive models of cytoskeletal organization. Here we show that the competing kinetics of bundle formation with the onset of dynamic arrest arising from filament entanglements and crosslinking determine the architecture of reconstituted actin networks formed with α-actinin crosslinks. Crosslink-mediated bundle formation only occurs in dilute solutions of highly mobile actin filaments. As actin polymerization proceeds, filament mobility and bundle formation are arrested concomitantly. By controlling the onset of dynamic arrest, perturbations to actin assembly kinetics dramatically alter the architecture of biochemically identical samples. Thus, the morphology of reconstituted F-actin networks is a kinetically determined structure similar to those formed by physical gels and glasses. These results establish mechanisms controlling the structure and mechanics in diverse semiflexible biopolymer networks. The spatiotemporal regulation of actin cytoskeleton organization is required for numerous eukaryotic cellular processes including adhesion, polarity, migration, division, endocytosis and intracellular trafficking [1] . Actin filaments (F-actin) are variably assembled by actin-binding proteins into a myriad of mesoscopic structures, including bundles of axially aligned filaments and meshworks of filaments crosslinked at high angles. The mechanics and dynamic properties of these different actin organizations are essential for supporting the physical and morphogenic aspects of distinct cellular processes. Understanding the biochemical and physical mechanisms regulating the assembly of actin-based structures is central to developing a quantitative understanding of cytoskeletal organization. Reconstituted actin networks provide the capability to isolate molecular and physical mechanisms underlying the self-assembly of actin-based structures. While the molecular architecture of actin crosslinking proteins can have an important role in the network morphology [2] , [3] , most actin crosslinking proteins such as α-actinin, filamin, fascin, fimbrin and scruin form a variety of actin structures, ranging from fine meshworks to networks of thick bundles [3] , [4] , [5] , [6] , [7] , [8] . It has been suggested that the morphology of crosslinked actin networks reflect thermodynamic equilibrium configurations similar to those observed in the isotropic-nematic phase transition of liquid crystals [9] , [10] , [11] , [12] , [13] . However, recent data suggest that reconstituted F-actin networks exhibit behaviours reminiscent of materials far-from-equilibrium, such as gels or glasses [14] , [15] . Thus, the extent to which the morphology of reconstituted actin networks reflects an equilibrium or non-equilibrium configuration is unknown. The lack of knowledge of parameters controlling the morphology of actin networks formed in vitro prevents the development of accurate models describing cytoskeletal organization in a complex, cellular environment. Here, we show that the morphology of reconstituted actin networks formed with α-actinin is determined by the competing effects of two processes intimately tied to actin polymerization kinetics: crosslinker-mediated bundling of F-actin and dynamic arrest of filament mobility. We demonstrate that bundle formation occurs only when the local microenvironment is predominately fluid, facilitating rotational and translational diffusion of filaments that permits their α-actinin-mediated bundle formation. Within a fluid microenvironment, the rate of bundle formation increases with the concentration of actin filaments and α-actinin, consistent with mass action kinetics. As actin polymerization proceeds, bundle formation is impeded concomitantly with arrested filament mobility. The onset of dynamic arrest is consistent with the formation of steric entanglements and crosslinking between filaments that occur when filament length is greater than the average filament spacing. As the onset of dynamic arrest controls the amount of time permissive to bundle formation, perturbations to F-actin assembly kinetics dramatically alters the density of bundles formed in biochemically identical samples. We develop a model to describe how the two kinetic processes of bundle formation and arrested filament mobility capture observed changes in bundle density. These results demonstrate that reconstituted actin network morphology reflects a kinetically determined structure far from thermodynamic equilibrium. These results have significant implications for the dynamic control of actin cytoskeletal organization in a crowded cytoplasm. Bundle assembly occurs over a narrow time interval To form F-actin networks crosslinked with smooth-muscle α-actinin, 5 μM monomeric actin was polymerized in the presence of varying concentrations of α-actinin and visualized after 1 h using confocal microscopy. Consistent with previous results, we observed different network morphologies over varying α-actinin concentrations [4] , [6] . At α-actinin concentrations c α <0.6 μM, a homogenous meshwork of entangled and crosslinked actin filaments formed ( Fig. 1 ). For c α =1.5–2.5 μM, a heterogeneous network of thick actin bundles embedded within a meshwork forms ( Fig. 1 ). When c α >2.5 μM, actin bundles become increasingly prevalent until the network is comprised almost entirely of thick actin bundles ( Fig. 1 ). While these varied morphologies of crosslinked actin networks have been well known for the past 25 years [3] , [4] , [5] , [6] , [7] , [8] , little is known about the underlying mechanisms of their assembly. 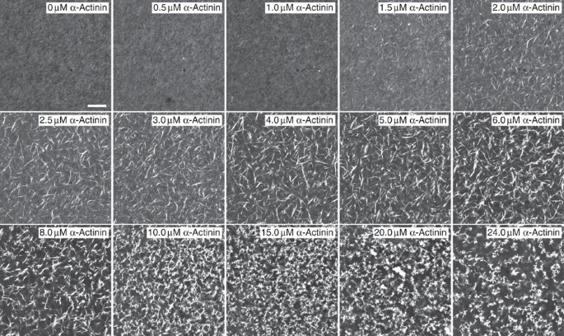Figure 1: Steady-state actin network architectures formed with varying concentrations of α-actinin images of fluorescent (Alexa 488) phalloidin-labelling of F-actin in networks formed by spontaneously assembling 5 μM G-actin in the presence of varying concentrations of α-actinin. Images were taken ~60 min after polymerization was initiated by the addition of salts. As α-actinin concentration is increased, the network architecture changes from single-filament meshwork (cα=0–1.0 μM) to a composite network (cα=1.5–3 μM), to a network of bundles (cα=4–10 μM), to a network that appears to be composed of very short and bright bundles of actin (cα>10 μM). Scale bar=30 μm. Figure 1: Steady-state actin network architectures formed with varying concentrations of α-actinin images of fluorescent (Alexa 488) phalloidin-labelling of F-actin in networks formed by spontaneously assembling 5 μM G-actin in the presence of varying concentrations of α-actinin. Images were taken ~60 min after polymerization was initiated by the addition of salts. As α-actinin concentration is increased, the network architecture changes from single-filament meshwork ( c α =0–1.0 μM) to a composite network ( c α =1.5–3 μM), to a network of bundles ( c α =4–10 μM), to a network that appears to be composed of very short and bright bundles of actin ( c α >10 μM). Scale bar=30 μm. Full size image To gain insight into the mechanism controlling the formation of actin bundles, we directly visualized their assembly using time-lapse confocal microscopy ( Fig. 2a , Supplementary Movie 1 ). Confocal imaging permits the acquisition of single thin (0.5 μm) optical sections up to 30 fps or a slow acquisition of full three-dimensional (3D) image stacks ( Supplementary Movies 2 , 3 and 4 ). Owing to rapid kinetics of network assembly, we focused our efforts on quantitative analysis of single-image planes. Approximately 60 s after initiating the polymerization of G-actin in the presence of 2 μM α-actinin, images of fluorescent phalloidin are uniform, indicating that little actin polymerization has occurred. By 135 s, short and highly mobile F-actin bundles appear. Subsequent interconnection and elongation of these structures, as well as nucleation of new filaments, forms an interconnected network of bundles by ~600 s that overlays well in a colour-combine image with the time point at 3660 s ( Fig. 2b ). Calculation of the static structure factor S ( q ) from these confocal images demonstrates that significant long-range order forms during network assembly and that this structure does not change significantly at times between 10–60 min ( Fig. 2c,d ). The lack of evolution in S ( q ) at long times suggests that we are operating in the strong crosslinking limit, where thermal fluctuations do not significantly disturb the network after its assembly. 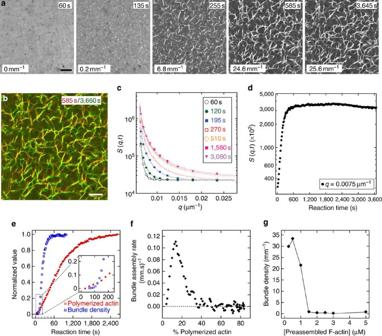Figure 2: Kinetics of bundle assembly and network formation. (a) Images of bundles formed by 5 μM actin and 2 μM α-actinin. Polymerization is initiated at time=0 s. Linear bundle density indicated on bottom left. (b) Colour-combine image of sample shown in part A att=585 s (red) and 3660 s (green). (c) Structure factor (S(q,t)) calculated for sample described in (a) at several representative time points during polymerization: 60 s (open black circles), 120 s (closed green circles), 195 s (closed blue squares), 270 s (open red squares), 510 s (open orange diamond), 1,560 s (closed magenta squares) and 3,060 s (closed purple inverted triangles). (d) Structure factorS(q,t) over time atq=0.0075 μm−1. (e) Pyrene assay (filled red circles) and bundle density (open blue squares) on networks of 5 μM actin with 2.0 μM α-actinin. Inset depicts the lag in bundle formation relative to actin polymerization. (f) Maximum bundle assembly rate versus F-actin concentration for data in (e). (g) Bundle density formed by mixing pre-polymerized F-actin with 0.6 μM α-actinin. Scale bars=30 μm. Data shown in (a–e) are of a single sample representative of results from at least 15 samples. Figure 2: Kinetics of bundle assembly and network formation. ( a ) Images of bundles formed by 5 μM actin and 2 μM α-actinin. Polymerization is initiated at time=0 s. Linear bundle density indicated on bottom left. ( b ) Colour-combine image of sample shown in part A at t =585 s (red) and 3660 s (green). ( c ) Structure factor ( S ( q , t )) calculated for sample described in ( a ) at several representative time points during polymerization: 60 s (open black circles), 120 s (closed green circles), 195 s (closed blue squares), 270 s (open red squares), 510 s (open orange diamond), 1,560 s (closed magenta squares) and 3,060 s (closed purple inverted triangles). ( d ) Structure factor S ( q , t ) over time at q =0.0075 μm −1 . ( e ) Pyrene assay (filled red circles) and bundle density (open blue squares) on networks of 5 μM actin with 2.0 μM α-actinin. Inset depicts the lag in bundle formation relative to actin polymerization. ( f ) Maximum bundle assembly rate versus F-actin concentration for data in ( e ). ( g ) Bundle density formed by mixing pre-polymerized F-actin with 0.6 μM α-actinin. Scale bars=30 μm. Data shown in ( a – e ) are of a single sample representative of results from at least 15 samples. Full size image Transverse line scans across fluorescent phalloidin images of F-actin solutions ( c α =0) revealed diffraction-limited peaks of variable intensity corresponding to ~1–10 actin filaments ( Supplementary Fig. S1a–c ). To distinguish bundles from individual filaments in crosslinked F-actin networks ( c α >0), we chose a minimum threshold intensity corresponding to a thickness of 15–30 filaments for bundle identification ( Supplementary Fig. S1 ). We then calculate the linear bundle density by counting the number of identified bundles per unit length; all results are robust to chosen threshold level ( Supplementary Fig. S1f ). Consistent with the qualitative observations in Fig. 2a and Supplementary Movie S1 , the bundle density increased very sharply from 0.2 mm −1 at 100 s to ~25 mm −1 at 585 s and remained constant thereafter ( Fig. 2e , blue squares). The slight decrease in linear bundle density after 600 s is due to photobleaching, as no evidence of bundle disassembly or large structural reorganization is observed ( Supplementary Movies 1 , 2 ). Thus, the formation of bundles occurs over a narrow time interval during the initial stages of network formation. Bundle formation occurs at low actin filament density To explore how the kinetics of bundle assembly is correlated to actin polymerization, we assessed the time courses of actin polymerization by pyrene fluorescence and bundle formation by fluorescence microscopy in identical samples. These two experimental techniques were completed within a few hours of each other and with the same stock of proteins. Actin polymerization is complete after ~2500 s, significantly longer than the time scale of bundle formation and dynamic arrest ( Fig. 2e ). In fact, the rate of bundle assembly is maximal when only 15% (0.75 μM) of the total actin is polymerized, and arrests when 40% (2 μM) of the actin is polymerized ( Fig. 2f ). Over half of the actin polymerization occurs after new bundle formation ceases ( Fig. 2e,f ). During this time, the intensity of existing bundles continues to increase, reflecting accumulation of F-actin into existing bundles ( Supplementary Fig. S1g ). F-actin also tends to accumulate in the meshwork surrounding the bundles during this time but is difficult to quantify through image analysis. Thus, the later stages of actin polymerization reinforce the existing network architecture, but do not contribute to new bundle formation. These data suggest that a high density of actin filaments inhibits bundle formation. To test this hypothesis, we mixed varying concentrations of pre-assembled actin filaments with 0.6 μM α-actinin and assessed the extent of bundling after 30 min. For F-actin concentrations below 0.5 μM, a high density of bundles forms ( Fig. 2g ). The extent of bundling sharply decreases as the F-actin concentration increases above 1.0 μM ( Fig. 2g ). Thus, a sufficiently high concentration of actin filaments can prevent bundle formation. Bundles form in a fluid-like microenvironment We speculated that the change in bundling rate is due to a change in the mechanical properties of F-actin's microenvironment, which may impede their rotational and translational mobility. In order to probe the mechanical properties of the microenvironment during actin network assembly, we included a low density of 1 μm-diameter polystyrene spheres to serve as probes for passive microrheology measurements [16] , [17] . We acquired bead images at 30 fps throughout the network assembly and used custom image processing software to calculate the mean-squared displacement (MSD) ‹Δ r 2 (τ)› over lag times τ much shorter than the time scales of bundle assembly, 0.1–5 s. The MSD of thermally driven tracer particles in a viscoelastic material can be fit to a power law in the form ‹Δ r 2 ( τ )›~ τ δ , where the scaling exponent δ reflects the viscoelasticity of the microenvironment ranging from δ =0 for an elastic solid to δ =1 for a viscous fluid [18] . Intermediate values of δ reflect a viscoelastic microenvironment with δ =0.5 indicating the transition between a viscoelastic fluid to viscoelastic solid [18] . A robust measure of the local mechanical environment yields an MSD scaling exponent that is independent of particle size [16] , [18] . The diffusive motion observed 60 s after the initiation of spontaneous polymerization of 5 μM actin in the presence of 3 μM α-actinin indicates a fluid microenvironment with a viscosity similar to that of water, ~1 mPa-s ( Fig. 3a , red circles and dashed line). However, anomalous diffusion is observed at later times, with δ decreasing from 0.8 to 0.2 over a period of 900 s ( Fig. 3a,b ), reflecting the formation of a predominately elastic actin gel. Actin filament polymerization significantly reduces the mobility of micron-sized probes as the MSD evaluated at τ =2 s decreases from 2 μm 2 to <0.25 μm 2 during the first 200 s of the reaction ( Fig. 3c ). The formation of bundles only occurs when the MSD is greater than 0.1 μm 2 ( Fig. 3c ). 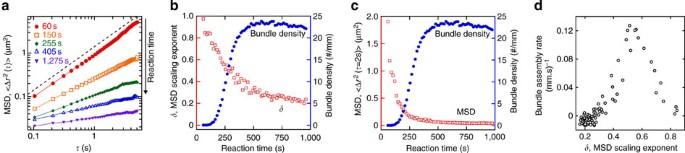Figure 3: Bundle assembly occurs in a predominately fluid microenvironment. (a) 2D MSD of 1-μm beads during assembly of a 5 μM G-actin and 3 μM α-actinin network at different times during polymerization: 60 s (red circles), 150 s (open orange squares), 255 s (green diamonds), 405 s (blue triangles) and 1,275 s (purple inverted triangles). The dashed line indicates diffusive motion. (b) The MSD scaling exponentδ(open red squares) and bundle density (filled blue circles) versus reaction time for the data in (a). (c) MSD evaluated atτ=2 s (open red squares) and bundle density (filled blue circles) versus reaction time for data obtained in (a). (d) Bundle assembly rate versus the MSD scaling exponentδ. Data from (a–d) are from a single sample representative of those obtained from at least ten independent samples. Figure 3: Bundle assembly occurs in a predominately fluid microenvironment. ( a ) 2D MSD of 1-μm beads during assembly of a 5 μM G-actin and 3 μM α-actinin network at different times during polymerization: 60 s (red circles), 150 s (open orange squares), 255 s (green diamonds), 405 s (blue triangles) and 1,275 s (purple inverted triangles). The dashed line indicates diffusive motion. ( b ) The MSD scaling exponent δ (open red squares) and bundle density (filled blue circles) versus reaction time for the data in ( a ). ( c ) MSD evaluated at τ =2 s (open red squares) and bundle density (filled blue circles) versus reaction time for data obtained in ( a ). ( d ) Bundle assembly rate versus the MSD scaling exponent δ . Data from ( a – d ) are from a single sample representative of those obtained from at least ten independent samples. Full size image Direct comparison of the bundle assembly rate with δ provides insight into the relationship between bundle formation and the mechanics of the local microenvironment. At earliest time points after initiation of actin polymerization, no bundles form and the microenvironment is predominantly fluid-like, reflecting a time with a very low F-actin density ( Fig. 3d ). Over time, the bundle assembly rate increases by 100-fold while δ decreases from 0.8 to 0.5, reflecting a time period where F-actin density rapidly increases and the local microenvironment is a viscoelastic fluid. When the F-actin density increases and the microenvironment becomes a viscoelastic solid ( δ <0.5), the bundle assembly rate sharply decreases ( Fig. 3d ). The formation of new bundles stops entirely when δ <0.3. To demonstrate that bead motions reflect changes in the mechanics of local environment, we confirm these results are independent of bead size ( Supplementary Fig. S2 ). These data indicate that as F-actin polymerization proceeds to form an interconnected gel with a solid-like microenvironment, bundle formation is dramatically impaired. Bundles only form when the microenvironment is predominately fluid. Accelerating actin dynamics abrogates bundle formation During spontaneous actin filament assembly, slow nucleation kinetics limit the polymerization rate at early times [19] . After the formation of a sufficient number of filament nucleates, the significantly faster filament elongation rate dominates and rapidly increases the polymer density. As we observed that bundles form at early times when filament nucleation limits the F-actin density, we sought to determine whether altering the nucleation kinetics affects bundle assembly. To bypass the slow nucleation step of F-actin assembly, we replaced varying fractions of monomeric actin with sheared actin filaments while maintaining constant G-actin and α-actinin concentration at 5 μM and 1 μM, respectively. These experiments allowed us to determine whether perturbations to the actin polymerization kinetics can alter network architecture. As the fraction of F-actin nucleates is increased from 0 to 10%, the bundle density at steady state increases from 21 mm −1 to 42 mm −1 ( Fig. 4a,b ). When the fraction of F-actin nucleates is increased beyond 25%, the density of high-intensity bundles decreases dramatically and only dim bundles below our threshold remain ( Fig. 4a,b ). 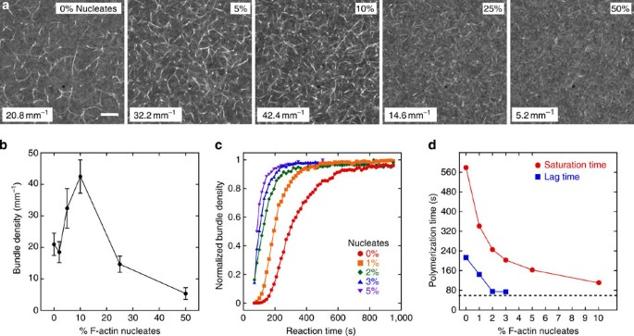Figure 4: Accelerating actin polymerization dynamics abrogates bundle formation. (a) Images of samples with identical concentrations of actin (5 μM) and α-actinin (1 μM) where the concentration of F-actin nucleates is increased from 0 to 50%. Linear bundle density indicated at the bottom left. Scale bar=30 μm. (b) Bundle density as a function of the percentage of F-actin nucleates for samples in (a). Error bars depict s.d. (n>15 fields of view) (c) Time course of normalized bundle assembly for samples with F-actin nucleates between 0–5% and identical concentrations of actin (5 μM) and α-actinin (2 μM). (d) Lag time (blue squares) and saturation time (red circles) for data in (c). Figure 4: Accelerating actin polymerization dynamics abrogates bundle formation. ( a ) Images of samples with identical concentrations of actin (5 μM) and α-actinin (1 μM) where the concentration of F-actin nucleates is increased from 0 to 50%. Linear bundle density indicated at the bottom left. Scale bar=30 μm. ( b ) Bundle density as a function of the percentage of F-actin nucleates for samples in ( a ). Error bars depict s.d. ( n >15 fields of view) ( c ) Time course of normalized bundle assembly for samples with F-actin nucleates between 0–5% and identical concentrations of actin (5 μM) and α-actinin (2 μM). ( d ) Lag time (blue squares) and saturation time (red circles) for data in ( c ). Full size image To explore how the bundle assembly kinetics are altered by changes in actin polymerization kinetics, we directly measured the bundle density from time-lapse images of F-actin during assembly of 5 μM actin in the presence of 2 μM α-actinin with varying concentrations of F-actin nucleates ( Supplementary Movie 5 ). The addition of F-actin nucleates facilitates the formation of bundles at earlier times ( Fig. 4c ), and the lag time before bundles begin to form at the start of the reaction decreases from 220 s to <60 s as the concentration of nucleates increases from 0 to 2% ( Fig. 4c,d ). In addition, the saturation time at which bundle density plateaus at a constant value also decreases from 560 s to 100 s ( Fig. 4c,d ). Thus, the time permissive to bundle assembly decreases from 340 s to <80 s as the concentration of nucleates increases from 0 to 10%. While a sufficiently high density of F-actin is necessary to form bundles, bundle assembly is impaired if filament nucleation proceeds too quickly. A similar response in the density of bundles to varied nucleate concentration is observed when c α =1.3 μM ( Fig. 5a,c ). When c α =0.6 μM, bundle density is sharply reduced once nucleates are introduced ( Fig. 5b,c ). Thus, the kinetics of actin polymerization dramatically change the architecture of samples constructed with identical concentrations of actin monomers and α-actinin crosslinks. 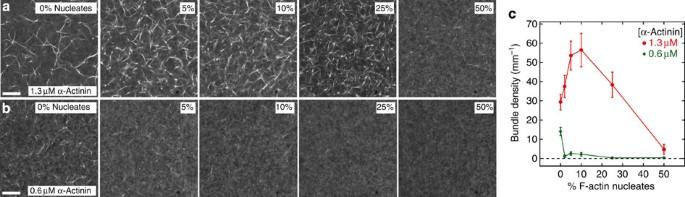Figure 5: Effect of nucleates on bundle density observed for different α-actinin concentrations. (a,b) Representative confocal images of steady-state architecture of actin networks formed with 5 μM actin and either (a)cα=1.3 μM α-actinin or (b)cα=0.6 μM α-actinin as the density of F-actin nucleates is increased from 0 to 50%. Scale bars=30 μm (c) The steady-state bundle density of samples described in (a) and (b). Figure 5: Effect of nucleates on bundle density observed for different α-actinin concentrations. ( a , b ) Representative confocal images of steady-state architecture of actin networks formed with 5 μM actin and either ( a ) c α =1.3 μM α-actinin or ( b ) c α =0.6 μM α-actinin as the density of F-actin nucleates is increased from 0 to 50%. Scale bars=30 μm ( c ) The steady-state bundle density of samples described in ( a ) and ( b ). Full size image α-actinin concentration determines bundle assembly rate The importance of α-actinin concentration in regulating the architecture of crosslinked F-actin networks has been well documented ( Fig. 1 ) [3] , [4] , [6] . As the ratio of α-actinin to actin increases, networks undergo a transition from single-filament meshwork to heterogeneous composite networks of bundles embedded into a single-filament meshwork and, ultimately, to a network of bundles ( Fig. 6a ). While previous work has speculated that this transition reflects changes in the equilibrium configuration of actin filaments with different crosslink densities [11] , [20] , our results suggest that the kinetics of bundle formation should be considered. 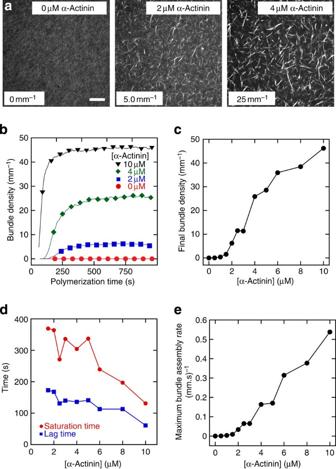Figure 6: α-Actinin concentration determines bundle assembly rate. (a) Images of 5 μM actin networks at steady state formed with [α-actinin]=0 μM, 2 μM and 4 μM. Linear bundle density indicated in bottom left. Scale bar=30 μm. (b) Time course of bundle assembly for representative α-actinin concentrations between 0–10 μM. (c) Bundle density versus α-actinin concentration. (d) Lag time (blue squares) and saturation time (red circles) for samples described in (a). (e) Maximum bundle assembly rate versus [α-actinin]. Figure 6: α-Actinin concentration determines bundle assembly rate. ( a ) Images of 5 μM actin networks at steady state formed with [α-actinin]=0 μM, 2 μM and 4 μM. Linear bundle density indicated in bottom left. Scale bar=30 μm. ( b ) Time course of bundle assembly for representative α-actinin concentrations between 0–10 μM. ( c ) Bundle density versus α-actinin concentration. ( d ) Lag time (blue squares) and saturation time (red circles) for samples described in ( a ). ( e ) Maximum bundle assembly rate versus [α-actinin]. Full size image We quantified the bundle density from a time-lapse image sequence of actin networks formed with concentrations of α-actinin ranging from 0 to 10 μM ( Fig. 6b , Supplementary Movie 6 ). Over this range, the steady-state bundle density increases from 0 to nearly 50 mm −1 ( Fig. 6c ). Neither the lag time nor the saturation time changes significantly as the α-actinin concentration increases from 1 to 5 μM ( Fig. 6d ), indicating that changes in the α-actinin concentration do not substantially alter the amount of time over which bundles form. Instead, we observe a 50-fold increase in bundle assembly rate as the concentration of α-actinin increases from 0 to 5 μM with a linear increase thereafter up to 10 μM ( Fig. 6e ). This suggests that increased α-actinin concentration serves primarily to enhance the rate of bundle assembly during the permissive time period at the initial stages of network assembly. The moderate reduction in both the lag and saturation times observed at the highest α-actinin concentrations indicates that α-actinin concentration may also have a secondary role in determining the time scales permissive to bundle formation, as has been suggested previously for the actin crosslinker filamin [21] . Kinetic model recapitulates experimental results We propose that the kinetics of actin filament polymerization dictate the amount of time over which bundle assembly is permitted. We found that bundle formation only occurs at dilute filament concentrations in a predominately fluid microenvironment. In 3D environments, the typical distance between filaments, ξ , is related to the sum of all filament and bundle concentrations c , ξ ~ c −1/3 . When the average filament length L is much smaller than ξ , actin filaments have rotational and translational freedom and the solution is predominately fluid [22] . In this regime, we speculate that bundle formation will be driven by the diffusion-limited rate of filament collisions, the rotational diffusion of filaments and the crosslink-mediated affinity of filaments ( Fig. 7a ). When the average filament length L is comparable to the distance between filaments ξ , filament overlaps result in reduced mobility due to steric entanglements as well as filament crosslinking. When L / ξ >1, impaired filament mobility results in a viscoelastic microenvironment on time scales shorter than relaxation times due to filament reptation or crosslink unbinding [22] , [23] . Thus, L / ξ ≈1 marks a transition from a microenvironment that is permissive to bundle assembly to one that is prohibitive ( Fig. 7a ). During the assembly of F-actin networks, both ξ and L vary with time as actin filaments nucleate and elongate. 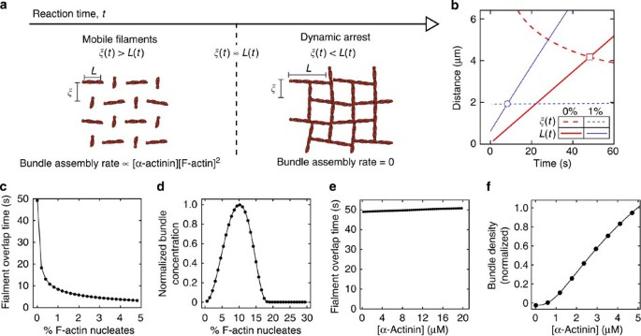Figure 7: Kinetic model recapitulates experimental results. (a) Schematic diagram of the stages of actin assembly during polymerization: the rate-limited bundle assembly reaction when filaments remain primarily mobile (ξ>L) and dynamically arrested, where bundle formation is inhibited by steric entanglements and high-angle crosslinks when filaments overlap (ξ<L). (b)ξ(t) andL(t) versus time during polymerization of 5 μM actin from monomers (red) and with 1% nucleates (blue). (c) Time to form filament overlaps versus density of F-actin nucleates. (d) Dependence of bundle density on F-actin nucleates. (e) Time to form overlaps as a function of [α-actinin]. (f) Bundle density as a function of [α-actinin]. In (b–d), F-actin nucleates have an initial length 0.8 μm and [α-actinin]=0.5 μM. Figure 7: Kinetic model recapitulates experimental results. ( a ) Schematic diagram of the stages of actin assembly during polymerization: the rate-limited bundle assembly reaction when filaments remain primarily mobile ( ξ > L ) and dynamically arrested, where bundle formation is inhibited by steric entanglements and high-angle crosslinks when filaments overlap ( ξ < L ). ( b ) ξ ( t ) and L ( t ) versus time during polymerization of 5 μM actin from monomers (red) and with 1% nucleates (blue). ( c ) Time to form filament overlaps versus density of F-actin nucleates. ( d ) Dependence of bundle density on F-actin nucleates. ( e ) Time to form overlaps as a function of [α-actinin]. ( f ) Bundle density as a function of [α-actinin]. In ( b – d ), F-actin nucleates have an initial length 0.8 μm and [α-actinin]=0.5 μM. Full size image To illustrate how different filament assembly conditions alter the amount of time where L / ξ < 1, we model the kinetics of filament growth based on previously established rate constants of actin nucleation and elongation [24] , [25] , [26] ( Supplementary Fig. S3 and Supplementary Methods ). The model consists of a system of coupled rate equations describing the concentrations of actin monomers, dimers, trimers and filaments with a specified average length, which account for the kinetics of filament nucleation and growth. This allows us to predict evolution of the filament length L ( Fig. 7b , solid lines) and concentration c as a function of time. Using this information, the average distance between filaments, or mesh size, is calculated by ξ ~ c −1/3 . For spontaneous filament nucleation, our model indicates that filament overlap occurs when L ≈ ξ ≈4 μm over 50 s ( Fig. 7b , red square). The addition of 1% of actin nucleates (trimers) virtually eliminates spontaneous nucleation, and filament overlap occurs for L ≈ ξ ≈2 μm at time ≈10 s ( Fig. 7b , dashed blue line). Increasing the fraction of added nucleates from 0 to 5%, the time to filament overlap is reduced by more than 10-fold ( Fig. 7c ). Thus, the addition of a small number of nucleates dramatically reduces the amount of time that the filaments remain freely mobile. We next supplement our model with chemical rate equations describing the irreversible coalescence of filaments into bundles at a rate proportional to the concentrations of α-actinin, filaments and bundles ( Supplementary Fig. S3–S5 and Supplementary Methods ). Further coalescence of bundles into larger bundles is also taken into account. In agreement with the above discussion, bundle formation is permitted only when L < ξ . This model recapitulates several key aspects of our experimental data. In the model, the total number of bundles shows a peak when 10% of the actin is added as F-actin nucleates ( Fig. 7d ), qualitatively similar to our experimental data ( Fig. 4b ). This can be understood by the competing effects of actin filament nucleates, which promote bundle assembly by increasing filament density while also accelerating the dynamic arrest. Furthermore, altering the α-actinin concentration in our simulations did not significantly reduce the time to form filament overlaps ( Fig. 7e ), which is consistent with the weak effect on the saturation time we observe when c α <6 μM ( Fig. 6d ). Finally, the model shows that increased α-actinin concentration enhances the rate of bundle assembly by a range of 50-fold ( Fig. 7f ), consistent with the observed rate increase ( Fig. 6e ). While this relatively simplistic kinetic model qualitatively captures many of our results, including more details on the nature of filament entanglements and bundling may yield quantitatively closer values and will be the subject of future theoretical work. We demonstrate that the morphology of networks formed by assembling actin filaments in the presence of the crosslinking protein α-actinin is determined by competing kinetics of bundle formation and arrest of filament mobility during actin filament polymerization. Instead of reflecting the thermodynamic equilibrium configuration of its components, the structures formed even by these simple reconstituted actin networks reflect a kinetically trapped metastable state that is determined during assembly. This is reminiscent of the ubiquitous kinetic constraints on structure and mechanics of physical gels and glasses [27] , [28] and consistent with recent observations [14] . As previous experiments only assessed the architecture of reconstituted actin networks at steady state, these kinetics effects have not been deeply considered despite a long history of studying the morphology of crosslinked F-actin networks [3] , [4] , [5] , [6] , [7] , [8] . The majority of efforts to understand the morphology of crosslinked actin networks have focused on the role of crosslinker-mediated aggregation of filaments with constant length [9] , [12] , [20] , [29] , and the energetic or kinetic constraints of bundling filaments within meshwork [30] , [31] , [32] . Our results are consistent with the recent experiments that demonstrate actin networks exhibit behaviours observed in materials far-from-equilibrium [14] , [15] . The potential role of actin polymerization kinetics in determining network architecture has been previously discussed [6] , [21] , [33] , but data supporting this behaviour have been lacking. Our data directly demonstrate that crosslinked actin networks are kinetically determined structures and identifies the role of actin nucleation and elongation kinetics in determining the time scale over which dynamic arrest occurs. By altering actin polymerization kinetics, the morphology of chemically identical samples can be modified. Thus, physical constraints arising from filament entanglements and crosslinking must be taken into account in models of actin cytoskeletal assembly even in remarkably simple reconstituted networks. Understanding the consequences of our results on the self-assembly of more complex cytoskeletal structures will be interesting to explore. Moreover, we speculate that these results will be generally applicable to studies of other biopolymer networks, including those formed from intermediate filaments, collagen, fibrin and microtubules. Numerous proteins that regulate the rates of actin filament nucleation and elongation are present in cells, which we speculate may have an important role in the formation of different cytoskeletal architectures. For instance, our work is consistent with observations that efficient nucleators such as Arp2/3 complex are prominent in meshworks while those that promote filament elongation such as vasodilator-stimulated phosphoprotein (VASP) and formins assist in bundle formation [19] , [34] . Moreover, the stability of in vitro meshworks after their assembly suggests that reorganization of even weakly crosslinked actin filament meshworks into bundles would be prevented under thermal motion in the absence of filament turnover. We speculate that significant reorganization in semidilute actin networks requires the action of actin severing or motor proteins to overcome effects of filament entanglement and crosslinking. It will be interesting to explore the competing roles of actin nucleators and severing proteins in controlling the morphology of in vitro networks. We speculate that these results will have a pronounced effect on the assembly of actin structures in dense and crowded environments, such as the cellular cytoplasm. Protein preparation Ca-ATP actin was purified from chicken skeletal muscle [35] . Gel-filtered actin was labelled on Cys-374 with pyrenyl iodoacetamide or Alexa Fluor 488 C5 maleimide (Invitrogen, Carlsbad, CA, USA) [36] . Immediately before each polymerization reaction, Ca-ATP-actin was converted to Mg-ATP-actin by adding 0.5 volumes of 0.6 mM EGTA and 0.15 mM MgCl 2 for 3 min at 25 °C. Extinction coefficients were used to determine protein concentrations of actin and pyrene-actin [35] . The concentration of AlexaFluor 488-labelled actin was measured by absorbance at 290 and 491 nm using the extinction of AlexaFluor 488 at 495 nm, ε 495 =71,000 M −1 cm −1 and a correction for AlexaFluor 488 absorbance at 290 nm A * 290 = A 290 −0.138· A 495 . Chicken smooth-muscle α-actinin ammonium sulphate precipitate (A9776, Sigma, St Louis, MO, USA) was diluted tenfold into 4 °C α-buffer (pH 7.6, 20 mM NaCl, 0.1 mM EDTA, 15 mM β-mercaptoethanol, 20 mM Tris-HCl and 10% glycerol) and dialysed in 12-kD MWCO tubing for 48 h at 4 °C against 1 l α-buffer, exchanging α-buffer three times at 12 h intervals. Sample was then bath sonicated at 4 °C for 1 h and centrifuged at 80,000 g for 2 h. The soluble α-actinin left in the supernatant is then transferred to an Amicon Ultra 30,000 MWCO filter unit (Millipore, Millerica, MA, USA), and concentrated to 10 μM and stored at 4 °C until use. The concentration of chicken smooth-muscle α-actinin was measured using the extinction coefficient estimated using ProtParam ( http://us.expasy.org/tools/ ) and the amino-acid composition: A 280 =128,500 M −1 cm −1 . In vitro network formation Actin networks were formed by mixing non-proteinaceous components first: glucose oxidase mix (4.5 mg ml −1 glucose, 0.5% β-mercaptoethanol, 4.3 mg ml −1 glucose oxidase and 0.7 mg ml −1 catalase), red fluorescent carboylate polystyrene FluoSpheres (Invitrogen), F-buffer (10 mM imidazole pH 7.0, 1 mM MgCl 2 , 50 mM KCl, 0.2 mM EGTA and 0.5 mM ATP), Ca-G-buffer(2 mM Tris pH 8.0, 0.2 mM ATP, 0.5 mM dithiothreitol, 1 mM sodium azide and 0.1 mM CaCl 2 ), α-buffer and 5% molar ratio of AlexaFluor 488-phalloidin (Invitrogen) to actin. We found that a 5% molar ratio of phalloidin to actin results in very little significant changes in the steady-state linear bundle density that was observed. α-Actinin was then added immediately following monomeric Mg-ATP actin to start the network assembly reaction. Each sample was mixed by pipetting up and down three times, loaded into its 5–10 μl sample chamber, sealed with Valap (1:1:1 by weight of vaseline, lanolin and parafin wax) and immediately transferred onto the confocal microscope for imaging. The time from the addition of monomeric actin to the start of imaging was between 60 and 80 s. Reaction time was measured relative to the time point when monomeric actin was added to the sample. Confocal microscopy and bundle analysis Sample chambers were constructed to dimensions of ~22 mm ( l )×1 mm ( w )×100 μm ( h ). All images were taken 50 μm above the bottom coverslip to minimize any edge effects that could affect bundle formation. Time-lapse images were taken at 15 s intervals with a ×20, 0.75 numerical aperture plan fluor objective. Spinning disk confocal images were collected with a CoolsnapHQ 2 camera (Photometrics, Tuscon, AZ, USA). We quantified bundle density in each frame with successive line scans in the x and y directions. A 63 mm of linear density was analysed in each frame. A peak detecting algorithm measured the height of local maxima above local minima along the line scan and marked these peaks as bundles if above a height threshold. These peaks are indicative of filamentous actin structures: single filaments, filament crossings or bundles. Dim peaks likely correspond to single filaments or points where a few filaments cross. The brighter a peak, the higher the probability that this peak identifies an actin bundle. The threshold for each sample was determined empirically by the peak analysis of a non-crosslinked 5-μM actin control network. The peak threshold was set relative to the average value in the image to a level that detects a linear bundle density <1 mm −1 . This was done to maintain as much sensitivity as possible for thin bundles, and eliminate the false identification of bundles due to multiple filaments crossing in the same confocal pixel. This analysis while robust for sensitively and accurately calculating linear bundle density is unable to obtain any information on the length distribution of such bundles. We estimate the minimum thickness for bundle detection using this method that is between 15 and 30 filaments. Pyrene assay Actin assembly was measured from the fluorescence of pyrene-actin with a Safire fluorescent plate reader [2] (Tecan, Durham, NC, USA) . Spontaneous assembly assays were performed on samples identical to those made for in vitro network formation, except with 10% pyrene-labelled Mg–ATP–actin. The in vitro network formation complementing each pyrene assay was assembled with the same stock of actin and actin-binding proteins, and were completed within 3 h of each other. A 15 μM mixture of pyrene-labelled and -unlabelled Mg–ATP–actin with ×100 anti-foam 204 (0.005%; Sigma) is added to the upper row of a 96-well non-binding black plate (Corning, Corning, NY, USA). All other components of the assay are added to the lower well: α-actinin, α-buffer, glucose oxidase mixture, ×10 F-buffer and Mg-G-buffer. Reactions were started by mixing lower wells with upper wells. Structure factor calculation The structure factor in Fig. 1 was calculated from the 2D Fourier Transform of a 1024×1024 pixel region taken from the center of each confocal slice in the time-lapse series of images used in the calculation of Fig. 1 . For each transform, a series of 225 radial line scans encompassing 360° were drawn out from the center of the transform and averaged over the radial distance. This calculation was repeated for each time step in the series and the results are shown in Fig. 1c,d . Microrheology We introduced 1-μm carboxylate-coated polystyrene beads, which bind stably and nonspecifically to actin filament networks [16] and allow us to probe the dynamics of the actin that within the network. Images obtained at 30 fps were recorded every 15 s between fluorescent images to obtain a time course throughout the assembly of the networks. The ~100 beads visible in each frame are tracked to subpixel accuracy via their centroids [37] . The ensemble-averaged MSDs of the particles at each time point during network assembly is calculated. Network formation with preassembled F-actin nucleates Preassembled actin nucleates were generated by polymerizing 10-μM Mg–ATP–actin in F-buffer for 1 h and shearing ×35 through a 26½ Gauge needle. The resulting actin nucleates were added after all the non-cytoskeletal components of the sample have been mixed. Immediately following this, the α-actinin and monomeric Mg–ATP–actin were added. The sample was then injected into the sample chamber, sealed and imaged as described before. How to cite this article: Falzone, T.T. et al . Assembly kinetics determine the architecture of α-actinin crosslinked F-actin networks. Nat. Commun. 3:861 doi: 10.1038/ncomms1862 (2012).